Probing relaxation times in graphene quantum dots Graphene quantum dots are attractive candidates for solid-state quantum bits. In fact, the predicted weak spin-orbit and hyperfine interaction promise spin qubits with long coherence times. Graphene quantum dots have been extensively investigated with respect to their excitation spectrum, spin-filling sequence and electron-hole crossover. However, their relaxation dynamics remain largely unexplored. This is mainly due to challenges in device fabrication, in particular concerning the control of carrier confinement and the tunability of the tunnelling barriers, both crucial to experimentally investigate decoherence times. Here we report pulsed-gate transient current spectroscopy and relaxation time measurements of excited states in graphene quantum dots. This is achieved by an advanced device design that allows to individually tune the tunnelling barriers down to the low megahertz regime, while monitoring their asymmetry. Measuring transient currents through electronic excited states, we estimate a lower bound for charge relaxation times on the order of 60–100 ns. Since the seminal work by Loss and DiVincenzo [1] , quantum dots (QDs) have been extensively tested as building blocks for solid-state quantum computation. Today, the most advanced implementations of QD qubits are realized in III/V heterostructures [2] , [3] , [4] . Nevertheless, the strong hyperfine interaction in these compounds poses fundamental limits to the spin coherence time, stimulating the search for alternative host materials, especially within the elements of group IV (ref. 5 ). In this context, graphene is a particularly promising candidate thanks to its low nuclear spin densities and weak spin–orbit interaction [6] , [7] , [8] . However, the gapless electronic band structure and the Klein tunnelling phenomenon [9] make it challenging to confine electrons electrostatically. This limitation can be circumvented by etching nanostructures in graphene, thus introducing a disorder-induced energy gap that allows the confining of individual carriers [10] , [11] , [12] , [13] , [14] , [15] , [16] , [17] . So far, excitation spectrum [18] , [19] , [20] , [21] , spin-filling sequence [22] and electron-hole crossover [23] have been studied in graphene QDs. However, these devices still lack the tunability of GaAs QDs, in particular with respect to the transparency of the tunnelling barriers, which hinders our ability to address the relaxation dynamics of individual quantum states experimentally. In this article, we present QDs with highly tunable barriers formed by long and narrow constrictions. This design is motivated by our recent study on the aspect ratio of graphene nanoribbons [17] , and it proved to be optimal to realize tunnelling barriers that can be tuned down to the low MHz regime. The enhanced control over the tunnelling barriers, combined with the information on their asymmetry provided by integrated charge detectors [24] , enable us to reach regimes where it is possible to investigate the excited states (ESs) relaxation dynamics via pulsed-gate transient current spectroscopy [25] , [26] . Our measurements indicate a lower bound for the charge relaxation time of about 60–100 ns. Device design and low-bias transport characterization Our devices consist of an etched graphene island (diameter, d =110 nm) connected to source and drain leads by long and narrow constrictions serving as tunnelling barriers ( Fig. 1a ). Two graphene nanoribbons, located symmetrically on each side of the island, can be used simultaneously as gates to tune the transparency of the barriers and as detectors sensitive to individual charging events in the dot [26] , [27] . The electrostatic potential of the QD is controlled by a central gate, on which a bias-tee mixes alternate current (AC) and direct current (DC) signals ( Fig. 1b ). This allows performing pulsed-gate experiments with the same gate used for DC control. The device is tuned by a back gate in the low charge-carrier density regime, where transport is dominated by Coulomb blockade effects [18] , [19] , [20] ( Supplementary Fig. S1a ). 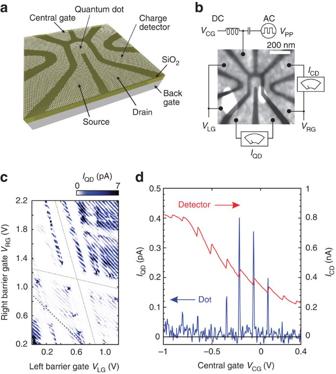Figure 1: Graphene QD device and low-bias transport measurements. (a,b) Schematic and scanning force micrograph of the measured device. The central island is connected to source and drain electrodes by two 40 nm wide and 80 nm long constrictions, whose transparency can be tuned by the voltage applied to the nearby nanoribbons (VLG,VRG). The nanoribbon on the right hand side is also used as a charge detector for the dot. The central gate is connected to a bias-tee mixing AC and DC signals. (c) Current through the dot as a function of the left and right gate voltagesVLG,VRG, recorded at a source-drain voltageVSD=−1.5 mV andVCG=0 mV. Here and in the following, the electron temperature isTe<100 mK, and the back gate voltage isVBG=34.6 V, corresponding to a Fermi level deep in the transport gap (Supplementary Fig. S1a). Different families of resonances can be identified in this measurement, which can either be attributed to the dot (features with relative lever arm 0.9; dotted line) or to localized states either in the left or right constriction (features with a relative lever arm of 5 and of 0.25, respectively; dashed lines). This indicates the possibility of tuning the transparency of the two constrictions independently, and controlling the current through the dot down to the sub-pA level by acting onVLG,VRG. (d) Simultaneous measurements of the current flowing through the dot and through the right nanoribbon as a function ofVCG. The bias voltage applied to the dot and to the nanoribbon areVSD=−1.5 mV andVCD=0.2 mV, respectively. Barrier-gate voltages areVLG=0.4 V andVRG=0 V. Figure 1: Graphene QD device and low-bias transport measurements. ( a , b ) Schematic and scanning force micrograph of the measured device. The central island is connected to source and drain electrodes by two 40 nm wide and 80 nm long constrictions, whose transparency can be tuned by the voltage applied to the nearby nanoribbons ( V LG, V RG ). The nanoribbon on the right hand side is also used as a charge detector for the dot. The central gate is connected to a bias-tee mixing AC and DC signals. ( c ) Current through the dot as a function of the left and right gate voltages V LG, V RG , recorded at a source-drain voltage V SD =−1.5 mV and V CG =0 mV. Here and in the following, the electron temperature is T e <100 mK, and the back gate voltage is V BG =34.6 V, corresponding to a Fermi level deep in the transport gap ( Supplementary Fig. S1a ). Different families of resonances can be identified in this measurement, which can either be attributed to the dot (features with relative lever arm 0.9; dotted line) or to localized states either in the left or right constriction (features with a relative lever arm of 5 and of 0.25, respectively; dashed lines). This indicates the possibility of tuning the transparency of the two constrictions independently, and controlling the current through the dot down to the sub-pA level by acting on V LG, V RG . ( d ) Simultaneous measurements of the current flowing through the dot and through the right nanoribbon as a function of V CG . The bias voltage applied to the dot and to the nanoribbon are V SD =−1.5 mV and V CD =0.2 mV, respectively. Barrier-gate voltages are V LG =0.4 V and V RG =0 V. Full size image The QD is first characterized by low-bias transport measurements ( Fig. 1c ) as a function of the voltage applied to the two side gates controlling the transparency of the barriers [18] . The optimized design of our device allows us to individually tune the tunnelling rates of both barriers (Γ L , Γ R ) over a wide range. By suppressing these rates we can access the sequential tunnelling regime, where the dot current exhibits approximately equally spaced Coulomb resonances as a function of the voltage V CG applied to the central gate, with peak currents up to a few hundred fA ( Fig. 1d , lower curve). A current of 200 fA corresponds to an overall dot transmission rate of Γ<1.25 MHz. In correspondence of each Coulomb peak, the current through the graphene nanoribbon on the right side of the QD shows characteristic sharp kinks ( Fig. 1d , upper curve), which indicate that the nanoribbon acts as a sensitive charge detector for the QD [27] , [28] . Excited states spectroscopy and charge sensing The addition energy of the dot and its ES spectrum are then probed by finite-bias spectroscopy. 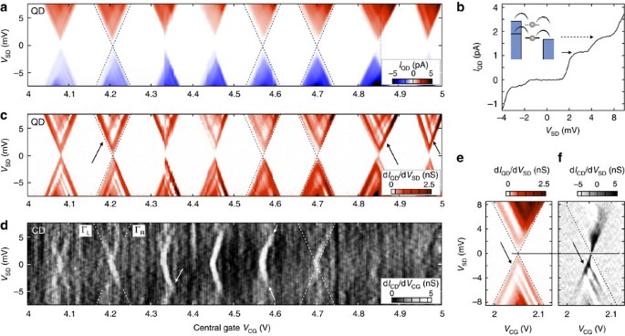Figure 2: Finite-bias ES spectroscopy and charge sensing. (a) Current through the QD as function ofVCGand the source-drain biasVSDin a regime of weak tunnel coupling to the leads; the dashed lines are guides to the eye indicating the edges of the Coulomb diamonds. (b) Line-cut at constantVCG=4.86 V, marked by a line in (a): the stepwise increase of the current is a signature of the discrete QD spectrum; the two well-defined plateaus correspond to the GS and the first ES entering the bias-window. (c) Differential conductance of the QD, dIQD/dVSD. Resonances parallel to both edges of the Coulomb diamonds, indicating transport through ESs, can be clearly seen. (d) Derivative of the charge-detector currentICDwith respect toVCG. Regions of high dICD/dVCGcorrespond to the onset of the transitions with the largest rate, thus providing information on the asymmetry of the tunnelling barriers. Note that this effect can be bias dependent (for example, the diamond centred onVCG≈4.45 V is more strongly coupled to the right lead forVSD>0 and to the left one forVSD<0) and it can be drastically influenced by the onset of transitions through ESs, as indicated by the appearance of kinks as those marked by the arrow. (e,f) Simultaneous measurements of the differential conductance of the dot dIQD/dVSD(e) and of the transconductance of the charge detector dICD/dVSD(f) in a regime of interest for pulsed-gate experiments. Figure 2a show the current and the differential conductance through the QD. These Coulomb diamond measurements give an estimate of the addition energy of the QD, E add ≈10.5 meV. In a simple disc-capacitor model, this corresponds to a QD diameter of 120 nm, in good agreement with the geometric size of our device. Clear signatures of transport through well-defined ESs can be already observed in the current (for example, see Fig. 2b ). They become even more evident in the differential conductance ( Fig. 2c ), from which we extract a level spacing of about Δ=1.5–2.5 meV. This is in agreement with the electronic single-particle level spacing given by meV, where N , the number of carriers on the dot, is assumed to be on the order of 10–20 (ref. 20 ). Figure 2: Finite-bias ES spectroscopy and charge sensing. ( a ) Current through the QD as function of V CG and the source-drain bias V SD in a regime of weak tunnel coupling to the leads; the dashed lines are guides to the eye indicating the edges of the Coulomb diamonds. ( b ) Line-cut at constant V CG =4.86 V, marked by a line in ( a ): the stepwise increase of the current is a signature of the discrete QD spectrum; the two well-defined plateaus correspond to the GS and the first ES entering the bias-window. ( c ) Differential conductance of the QD, d I QD /d V SD . Resonances parallel to both edges of the Coulomb diamonds, indicating transport through ESs, can be clearly seen. ( d ) Derivative of the charge-detector current I CD with respect to V CG . Regions of high d I CD /d V CG correspond to the onset of the transitions with the largest rate, thus providing information on the asymmetry of the tunnelling barriers. Note that this effect can be bias dependent (for example, the diamond centred on V CG ≈4.45 V is more strongly coupled to the right lead for V SD >0 and to the left one for V SD <0) and it can be drastically influenced by the onset of transitions through ESs, as indicated by the appearance of kinks as those marked by the arrow. ( e , f ) Simultaneous measurements of the differential conductance of the dot d I QD /d V SD ( e ) and of the transconductance of the charge detector d I CD /d V SD ( f ) in a regime of interest for pulsed-gate experiments. Full size image Important information on the asymmetry of the barriers can be inferred by plotting d I CD /d V CG (ref. 24 ), where I CD is the current flowing through the charge detector (see Fig. 2d ). Regimes where the coupling to the leads is comparable in magnitude are characterized by the appearance of regions of high d I CD /d V CG in correspondence of both edges of a Coulomb diamond ( cf. the diamond centred around V CG ≈4.2 V). Vice versa, regimes where one of the tunnel barriers is dominating are signalled by a strongly one-sided d I CD /d V CG ( cf. diamond centred around V CG ≈4.45 V). This knowledge permits to identify regimes where the relaxation dynamics of the ESs can be investigated by pulsed-gate spectroscopy [25] , [26] . This technique requires in fact the pulse rise time ( τ rise ) to be the fastest timescale in the system, that is, both tunnel rates (Γ L , Γ R ) need to be much slower than τ rise −1 . To ensure that this condition is satisfied, we tune the dot into a low current regime where the tunnelling barriers are roughly equal. Conductance measurements in such a regime are shown in Fig. 2e . Note that the charge detector is such a sensitive electrometer that QD ESs can be clearly resolved in the differential transconductance d I CD /d V SD ( Fig. 2f ). Pulsed-gate spectroscopy and transient currents To investigate the relaxation dynamics of ESs in the graphene QD, we employ a pulsed-excitation scheme similar to the one introduced by Fujisawa et al . [25] , [26] , [29] . The basic idea is to probe transient phenomena in a QD by measuring the averaged DC-current flowing through the system in the presence of a small (fixed) bias voltage V SD and of a square voltage-pulse applied to one of the gates (see Fig. 3a ). The crucial requirement is that the rise time of the pulse has to be much shorter than the inverse of the tunnel rates, so that the occupation of the QD cannot follow adiabatically the change of the potential and, when the pulse-level switches from high to low (or vice versa), the system is brought in a state of non-equilibrium. If the frequency of the pulse is low (100 kHz in Fig. 3b ), the square-wave modulation of the gate voltage results simply in the splitting of the Coulomb resonance into two peaks [30] . These peaks stem from the QD ground state (GS) entering the bias-window at two different values of V CG, one for the lower pulse-level (A), and one for the upper one (B). At larger frequencies (800 kHz in Fig. 3d ), together with the splitting there is an additional broadening of the peaks. The situation changes dramatically at higher frequencies (from a few to tens of MHz), where a number of additional peaks appear, due to transient transport through QD ESs (see Fig. 3e ). Each of these additional resonances corresponds to a situation in which the QD levels are pushed well outside the bias-window in the first half of the pulse, and then brought into a position where transport can occur only through the ESs in the second one, see Fig. 3f . No current can flow in any of these two configurations in the stationary state. However, in the second half of the pulse electrons can tunnel from one lead to the other via the ES, as long as the GS remains unoccupied (see Supplementary Fig. S2 ). Once the GS gets filled, either because of tunnelling from the leads or relaxation from the ES, transport is blocked. The blockade is released by returning the pulse-level to its initial value. In these conditions, a square-wave modulation of the gate voltage results in a train of short current pulses, which can be resolved in our DC-current measurements only if the frequency of the pulse is higher than the characteristic rate γ of the blocking processes. The lowest frequency at which signatures of transport through ESs emerge provides, therefore, an upper bound for γ . 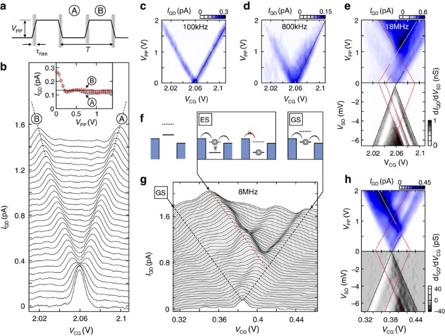Figure 3: Pulsed-gate spectroscopy of ESs. (a) Sketch of the pulse scheme employed in the measurements presented in this figure (duty-cycle 50%). Low and high pulse-level are labelled A and B, respectively. (b) Current through the dot while applying a 100-kHz pulse. Different lines correspond toVPPbeing varied from 0 to 1.4 V in steps of 50 mV (lines offset by 0.05 pA for clarity). Here and in the followingVSD=−1.5 mV. Increasing the amplitude of the pulse, the Coulomb peak splits in two resonances that shift linearly withVPPand whose height is approximately half the one of the original peak (see inset). (c,d) Colour-scale version of the data shown inb. Indthe pulse frequency is 800 kHz. (e) Upper panel: same measurement as (b–d), at a higher frequency of 18 MHz. Together with the GS splitting, a number of additional resonances can be seen, corresponding to transient currents through ESs. The level spacing extracted from this measurement coincides with the one given by DC finite-bias measurements (lower panel, same data as inFig. 2e). The dashed lines are guides to the eye. (f) Schematic of transport via GS, ES and, on the left, of a possible initialization stage. (g) Measurement similar to the ones shown inb, but for a different Coulomb resonance. Here the pulse frequency is 8 MHz,VSD=−1 mV, andVPPis varied from 0 to 2 V in steps of 25 mV (traces offset by 0.02 pA). (h) Same data set as ingand comparison with the corresponding DC measurement, showing excellent agreement between the ESs level spacing extracted from pulsed-gate and finite-bias spectroscopy. Figure 3: Pulsed-gate spectroscopy of ESs. ( a ) Sketch of the pulse scheme employed in the measurements presented in this figure (duty-cycle 50%). Low and high pulse-level are labelled A and B, respectively. ( b ) Current through the dot while applying a 100-kHz pulse. Different lines correspond to V PP being varied from 0 to 1.4 V in steps of 50 mV (lines offset by 0.05 pA for clarity). Here and in the following V SD =−1.5 mV. Increasing the amplitude of the pulse, the Coulomb peak splits in two resonances that shift linearly with V PP and whose height is approximately half the one of the original peak (see inset). ( c , d ) Colour-scale version of the data shown in b . In d the pulse frequency is 800 kHz. ( e ) Upper panel: same measurement as ( b – d ), at a higher frequency of 18 MHz. Together with the GS splitting, a number of additional resonances can be seen, corresponding to transient currents through ESs. The level spacing extracted from this measurement coincides with the one given by DC finite-bias measurements (lower panel, same data as in Fig. 2e ). The dashed lines are guides to the eye. ( f ) Schematic of transport via GS, ES and, on the left, of a possible initialization stage. ( g ) Measurement similar to the ones shown in b , but for a different Coulomb resonance. Here the pulse frequency is 8 MHz, V SD =−1 mV, and V PP is varied from 0 to 2 V in steps of 25 mV (traces offset by 0.02 pA). ( h ) Same data set as in g and comparison with the corresponding DC measurement, showing excellent agreement between the ESs level spacing extracted from pulsed-gate and finite-bias spectroscopy. Full size image Probing relaxation times A more accurate estimate of the relaxation time of the ESs can be obtained with a different pulse scheme (see Fig. 4a ), where T A is varied while keeping T B and V PP fixed [25] , [26] , [31] . Such a measurement is shown in Fig. 4b for the same Coulomb resonance investigated in Fig. 3b–e . The two outermost peaks correspond to transport via the dot GS when this is in resonance with the bias-window during T A (right peak) and T B (left peak). The inner peak results from transport via an ES, as indicated in the scheme sketched in Fig. 4c . For each of these peaks, we estimate the average number of electrons tunnelling through the device per cycle ‹ n ›= I ( T A + T B )/ e . 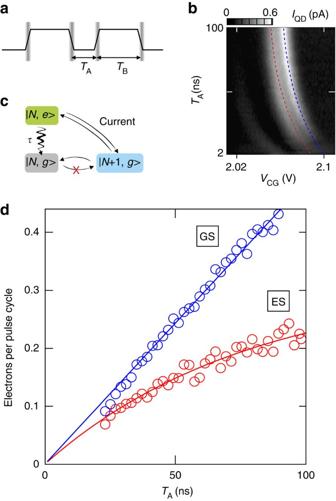Figure 4: Transient current through ESs. (a) Pulse scheme used to study transient currents through ESs: timeTBis fixed, while timeTAis varied. (b) Current through the QD as a function ofVCGandTAforVSD=−1 mV,VPP=0.9 V,TB=30 ns. All lines are bent due to a parasitic effect of the bias-tee adding a duty-cycle dependent DC-offset toVCG. Dashed lines indicate the peaks due to transport via GS (blue) and ES (red), further investigated ind. (c) Schematic of the transitions occurring duringTAfor the central peak inb. |N,g› (|N,e›) indicates the ground (excited) state of the dot withNexcess electrons. The transition |N,g›→|N+1,g› is not energetically allowed in the range of values used forVSDandVCGduringTA, and so |N,g› is an ‘absorbing’ state. At the beginning of each cycle, the dot is initialized in the state withN+1 electrons duringTB(not shown). (d) Average number of electrons transmitted per cycle through GS (blue circles) and ES (red circles), as a function of the pulse lengthTA. Data are extracted from the peaks shown inb, solid lines represent linear and exponential fit to the experimental data (1/γ=78 ns,nsat=0.313). Figure 4d shows the number of electrons transmitted via the GS (blue) and via the ES (red) as a function of the pulse length T A . While the first one increases linearly with T A , the second tends to saturate, indicating a transient effect. Fitting this data set with n ( T A )= n sat [1-exp(− γ T A )], where n sat is the saturation value for long T A (ref. 25 ), we extract the characteristic rate of the blocking processes γ =12.8 MHz. As both tunnelling and relaxation lead to the occupation of the GS, γ is approximately given by γ ~Γ+1/ τ , where τ is the intrinsic relaxation time of the ES and Γ the characteristic tunnelling rate. This in turn gives a lower bound τ >78 ns for the lifetime of the QD ES. By studying further electronic ESs with energies in the range of 1.7–2.5 meV (see Supplementary Fig. S3–S5 ), we estimate a lower bound for the relaxation time in the range 60–100 ns. Figure 4: Transient current through ESs. ( a ) Pulse scheme used to study transient currents through ESs: time T B is fixed, while time T A is varied. ( b ) Current through the QD as a function of V CG and T A for V SD =−1 mV, V PP =0.9 V, T B =30 ns. All lines are bent due to a parasitic effect of the bias-tee adding a duty-cycle dependent DC-offset to V CG . Dashed lines indicate the peaks due to transport via GS (blue) and ES (red), further investigated in d . ( c ) Schematic of the transitions occurring during T A for the central peak in b . | N , g › (| N , e ›) indicates the ground (excited) state of the dot with N excess electrons. The transition | N , g ›→| N +1, g › is not energetically allowed in the range of values used for V SD and V CG during T A , and so | N , g › is an ‘absorbing’ state. At the beginning of each cycle, the dot is initialized in the state with N +1 electrons during T B (not shown). ( d ) Average number of electrons transmitted per cycle through GS (blue circles) and ES (red circles), as a function of the pulse length T A . Data are extracted from the peaks shown in b , solid lines represent linear and exponential fit to the experimental data (1/ γ =78 ns, n sat =0.313). Full size image The experimentally observed relaxation timescale is likely related to the lifetime of charge excitations, which is limited by electron–phonon interaction. Interestingly, the extracted charge relaxation times are a factor 5–10 larger than what has been reported in III/V QDs [25] , [26] , [31] , [32] . This might be a signature of reduced electron–phonon interaction in sp 2 -bound carbon, where piezoelectric phonons are absent. To test this hypothesis, we perform a preliminary estimate of relaxation times in graphene QDs based on simplified assumptions for the QD and the phonon density of states (see Methods). Assuming that the coupling to longitudinal acoustic (LA) phonons via the deformation potential is the most dominant relaxation mechanism [33] , we obtain relaxation times in the range 40–400 ns for an ideal circular graphene QD with 110 nm diameter (see Supplementary Fig. S6 ). This is in reasonable agreement with the lower bound for the relaxation time τ extracted from the pulsed-gate measurements. It should, however, be kept in mind that these estimates are based on a very simplified model. More realistic calculations should take into account the effects of the destroyed graphene lattice, which breaks the A-B lattice symmetry and leads to a phonon density of states that is strongly dependent on the exact shape of the QD itself. In summary, in this article we experimentally address the dynamics of ESs in graphene QDs. This is achieved by employing an innovative device design that allows realizing highly tunable graphene QDs, suitable for investigations with pulsed-gate spectroscopy. Measuring transient currents through ESs, we obtain a lower bound of 60–100 ns for the relaxation time of electronic excitations. Our work indicates a clear strategy of optimizing the sample design for pulse-gate experiments, and represents a fundamental step towards the investigation of spin life-times and coherence times in graphene QDs. Device fabrication The sample is fabricated by mechanical exfoliation of natural bulk graphite. Graphene flakes are transferred to highly doped silicon substrates with a 295-nm silicon oxide top-layer. Single-layer flakes are selected via Raman spectroscopy. The Raman spectrum of the measured graphene flake shows a 2D-peak with full width at half maximum (FWHM) of 34 cm −1 ( cf. Supplementary Fig. S1b ). The peak amplitude of the 2D-line is almost twice as high as the G-line, proving that the flake is one monolayer thick [34] . The flake is then patterned by electron beam lithography, followed by Ar/O 2 reactive ion etching. A second electron beam lithography and evaporation (5/50 nm Cr/Au) step is performed to create source and drain electrodes and gate contacts on the graphene device. Transport measurements All measurements are performed in a dilution refrigerator, at a base temperature of ~20 mK. We use home-built low-noise DC amplifiers (amplification factor of the order 10 8 , bandwidth <1 kHz, integration time 200 ms) to measure currents with a precision better than 50 fA. For the pulsed-gate experiments, we use the arbitrary waveform generators Tektronix AWG520 and Tektronix AWG7082C, and the bias-tee Anritsu K251 to mix AC and DC signals on the central gate. Two attenuation stages (10 dB attenuator at room temperature and 20 dB attenuator at 4 K) and impedance mismatch reduce the amplitude of the pulse at the sample by a factor 15.8 (24 dB) with respect to the one produced by the generator. The pulse shape remains, however, almost unperturbed ( cf. Supplementary Fig. S7 ). The rise time detected close to the sample is about 250–300 ps. Measurements were performed in two different devices with the same lithographic design. Both devices show similar behaviour. Data from the second sample are shown in the Supplementary Fig. S8 . Estimating relaxation times in graphene QDs A preliminary estimate of charge relaxation time τ in graphene QDs can be obtained in terms of Fermi’s golden rule , by making some simplified assumptions on the electron-phonon coupling Hamiltonian H el−ph and the shape of the electronic wave functions Ψ i and Ψ f . To this end, we model the graphene QD as a circular disc of radius R =55 nm confined by an infinite mass term [35] . The dot states are then eigenfunctions of the following Hamiltonian: , where the first term on the right hand side is the Dirac-like graphene Hamiltonian and the second one includes a mass-related potential energy term V ( r ) ( κ is here the valley index), which is zero inside the QD but tends to infinity towards the edges, that is, V ( r )=0 for r < R and V ( r )→∞ for r ≥ R (refs 35 , 36 ). The wave functions of such a Hamiltonian are given by: Where J m ( x ) are Bessel functions of the first kind, are normalization constants and k n are the solutions of the equation J m ( kR )= κJ m +1 ( kR ) ( 36 ). Assuming the coupling to the LA phonon mode via deformation potential to be the dominant cause of relaxation (see Supplementary Note ), and that at the low temperature of the experiment the phonons are in their ground state, the electron-phonon coupling Hamiltonian take the form [37] where D is the deformation potential, A the area of the graphene QD, ρ =7.5 × 10 −7 kg m −2 the mass density and v s =2 × 10 4 m s −1 the sound velocity of the LA mode. The creation operator describes the emission of one phonon. With these ingredients, the inverse relaxation time can be written as where and q 0 =Δ/ v s , is the wave vector of a phonon whose energy matches the QD level spacing Δ. This expression can be computed numerically and in Supplementary Fig. S6 , we show the calculated relaxation times τ as function of the level spacing Δ. We find that for a level spacing in the range of 1.5–2.5 meV, coupling to LA phonons results in relaxation times on the order of 40–400 ns, in reasonable agreement with our experimental findings. How to cite this article: Volk, C. et al . Probing relaxation times in graphene quantum dots. Nat. Commun. 4:1753 doi: 10.1038/ncomms2738 (2013).